Highly emissive excitons with reduced exchange energy in thermally activated delayed fluorescent molecules Unlike conventional thermally activated delayed fluorescence chromophores, boron-centered azatriangulene-like molecules combine a small excited-state singlet-triplet energy gap with high oscillator strengths and minor reorganization energies. Here, using highly correlated quantum-chemical calculations, we report this is driven by short-range reorganization of the electron density taking place upon electronic excitation of these multi-resonant structures. Based on this finding, we design a series of π-extended boron- and nitrogen-doped nanographenes as promising candidates for efficient thermally activated delayed fluorescence emitters with concomitantly decreased singlet-triplet energy gaps, improved oscillator strengths and core rigidity compared to previously reported structures, permitting both emission color purity and tunability across the visible spectrum. The discovery of purely organic thermally activated delayed fluorescence (TADF) materials, with its premise to break the spin statistical bottleneck of 25% internal quantum efficiency without the requirement of rare noble metal emitters, has prompted a paradigm shift in the design of emitter materials for use in organic light-emitting diodes (OLEDs) [1] . TADF is rooted in a thermally promoted reverse intersystem crossing (RISC) process enabling upconversion of triplet excitons into emissive singlet excitons, which otherwise would be lost through non-radiative pathways. One key property TADF molecules should fulfill for efficient RISC is a small energy gap between the lowest singlet and triplet excited states Δ E ST (usually < 0.2 eV), so that delayed fluorescence can be thermally activated at room temperature (though exceptions to this general rule exist that involve higher-lying triplet states) [2] . The most widely applied design strategy so far is based on molecules featuring weakly coupled and spatially separated donor (D) and acceptor (A) moieties. This motif sustains charge-transfer (CT) excitations with small exchange interactions and correspondingly small Δ E ST compared to localized excited states [3] , [4] , [5] . However, this approach suffers from a number of drawbacks that directly reflect the nature of the emissive excited state. In particular, achieving high photoluminescence quantum yields (PLQY) and color purity in conventional TADF molecule-based OLEDs has been challenging thus far [6] , [7] , [8] , [9] . As a consequence of their dominant CT character, the singlet electronic excitations in these molecules often display fairly small radiative emission cross-sections (oscillator strengths, f osc ). Hence, high PLQY in these materials is only possible through efficient suppression of non-radiative decay processes. Moreover, charge-transfer excitations are usually accompanied by large structural reorganization, associated with conformational degrees of freedom in D-A molecular architectures, leading to broad emission spectra. Yet, such conformational gating effects also feed small admixtures of local (covalent) excited-state character into (primarily triplet) CT (ionic) excitations, prompting the needed spin-orbit interaction that mediates spin conversion [10] , [11] , [12] , [13] . Thus, designing optimally performing TADF compounds in this scenario relies on the necessarily delicate balance between antagonistic effects. A notable departure from the usual strategy has recently been proposed by Hatakeyama et al. [6] , [7] , [14] who designed TADF emitters as triangulene cores incorporating ortho -substituted boron and nitrogen atoms to promote multiple resonance effects (see chemical structures in Fig. 1 and resonant structures in Supplementary Fig. 5 ). Unlike conventional D-A architectures, these boron-centered azatriangulenes yield concomitantly narrow emission spectra (full-width at half-maximum = 28 nm), relatively large f osc (~0.2 for both DABNA-1 and 2 ) and small Δ E ST (~0.15 eV for DABNA-1 and 0.21 for 2 ) values. OLEDs with high maximum external quantum efficiencies (EQE max ) of 13.5% and pure blue emission [CIE coordinates of (0.13, 0.09] for DABNA-1 were demonstrated. In marked contrast with experiment, recent publications [5] , [15] , [16] reported Time-Dependent Density Functional Theory (TD-DFT) Δ E ST predictions in the range 0.4–0.6 eV depending on functional, largely overestimating the experimental values. Based on these TD-DFT calculations, two mechanistic pictures for TADF in boron-centered azatriangulenes molecules have been put forward: Lin et al. [15] claimed that RISC occurs directly from T 1 to S 1 while Northey et al. advanced that RISC involves an intermediate higher-lying triplet state T 2 [16] . Fig. 1 Evidence for short-range charge transfer in boron-centered azatriangulene molecules. a Chemical structures and b difference density plots of DABNA-1 and 2 (summing over the two doubly degenerated S 1 states, see Supplementary Fig. 4 ). Yellow (blue) color indicates increased (decreased) electron density upon S 0 -S 1 excitation Full size image Here, by scrutinizing the nature of the lowest electronic excitations in these molecules, we propose a new paradigm for TADF that builds on the concept of short-range charge-transfer illustrated in Fig. 1 . While long-distance charge separation in multichromophoric D-A systems reduces Δ E ST at the expense of f osc , we show that boron-centered azatriangulenes undergo a large but local spatial reorganization of the electronic density in the excited states, which significantly lowers the exchange energy while maintaining high overlap between wavefunction tails and therefore high f osc transitions, together with small structural relaxation energies. Based on these results, we propose analogs that we hope will lead to high performance TADF emitters in OLED devices. Origin of small Δ E ST in DABNA molecules We start our analysis with DABNA-1 [6] . Irrespective of the choice of the DFT functional and the use (or not) of the Tamm-Dancoff approximation, all our TD-DFT calculations yield erroneously large Δ E ST values (e.g., 0.56 eV at B3LYP level), in line with refs. 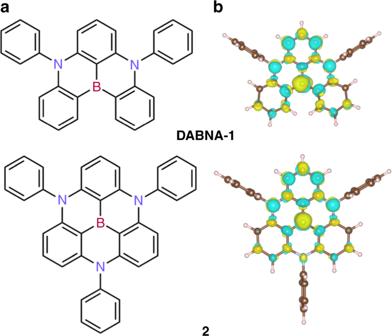Fig. 1 Evidence for short-range charge transfer in boron-centered azatriangulene molecules.aChemical structures andbdifference density plots ofDABNA-1and2(summing over the two doubly degenerated S1states, see Supplementary Fig.4). Yellow (blue) color indicates increased (decreased) electron density upon S0-S1excitation [6] , [15] , [16] (see Supplementary Table 1 ). The use of tuned range-separated functionals does not help either. By varying the amount of Hartree-Fock-like exchange in the functional, we observe a smooth decrease of Δ E ST that reaches a more reasonable 0.25 eV with pure semilocal models (e.g., LDA), but at the cost of an unphysical delocalization of the electronic density over the outer phenyl rings (Supplementary Fig. 1 ). The discrepancy between experiment and theory has more fundamental grounds, as we discovered by running higher-level Spin-Component Scaling second-order approximate Coupled-Cluster (SCS-CC2) calculations with the def2-TZVP basis set (see SI for further details on these calculations). In contrast to TD-DFT, SCS-CC2 calculations on DABNA-1 and compound 2 provide (vertical, i.e., based on ground-state geometry) Δ E ST values in excellent agreement with experiments, Table 1 . Despite relatively small Δ E ST values (<0.2 eV), the lowest singlet electronic excitation in these molecules is strongly dipole-allowed with a f osc of 0.31 in DABNA-1 and (summing over the two degenerated singlet excited states arising from the C 3V -symmetry) 0.26 in 2 . Most interestingly, similar Δ E ST values were obtained for vertical and adiabatic (fully relaxed) excitations, owing to modest nuclear reorganization energies in the S 1 state (0.12 eV and 0.10 eV for DABNA-1 and molecule 2 , respectively, Table 1 ), which should ensure narrow singlet emission as an added virtue. Table 1 Excited state properties Full size table The origin for the unusual electronic properties of these molecules is best pictured by difference density plots for the S 0 -S 1 and S 0 -T 1 excitations, calculated at the SCS-CC2 level and shown in Fig. 1b for DABNA-1 (cf. Supplementary Fig. 1 ). These plots reveal a remarkably homogenous short-distance reshuffling of the electronic density upon excitation that yields spatially alternating hole-rich and electron-rich regions. The density reorganization is partly shaped by second-order electronic correlation effects (Supplementary Fig. 2 ) and thus, not surprisingly, cannot be fully captured at the (one-electron) TD-DFT level. To elucidate further the origin for the small Δ E ST in DABNA-1 and 2 , it is instructive to analyze the results obtained for fragments (labeled fr1–fr5 in Fig. 2a ) extracted from the parent molecules. Close inspection of the differential density plots for both singlet and triplet excitations show the same alternating pattern as the one observed for DABNA-1 , yet with an increasing spreading in space as the fragment becomes larger and/or more conjugated, Fig. 2b . This effect can be quantitatively assessed by computing the CT delocalization volume (see Supplementary Information "Difference density plots" section for computational details). 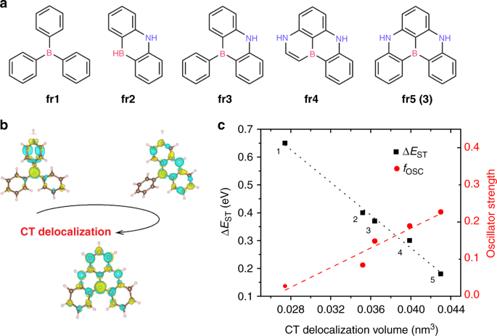Fig. 2 Charge transfer delocalization helps in decreasing the singlet-triplet energy gap and increasing the oscillator strength.aChemical structures of DABNA-1 fragments.bDifference density plots computed for selected fragments froma.cΔEST(black squares) and oscillator strengths,fosc(red dots) as a function of CT delocalization volume for the selected set of fragments Figure 2c shows strong linear correlations ( R 2 = 0.99) between both Δ E ST or f osc and the CT volume, with more extended systems providing, remarkably, smaller Δ E ST and larger f osc . The trend is in fact reminiscent of the behavior of localized (covalent) excitations in conjugated materials, where the exchange energy measured/calculated in polymer chains is usually significantly smaller than that in the parent small molecules [17] . Fig. 2 Charge transfer delocalization helps in decreasing the singlet-triplet energy gap and increasing the oscillator strength. a Chemical structures of DABNA-1 fragments. b Difference density plots computed for selected fragments from a . c Δ E ST (black squares) and oscillator strengths, f osc (red dots) as a function of CT delocalization volume for the selected set of fragments Full size image Highly emissive molecules with small Δ E ST The most striking feature arising from Fig. 2c is that while CT delocalization triggers a large decrease in Δ E ST from fr1 (0.65 eV) to fr5 (0.18 eV), the lowest excitation f osc strength instead increases along the same sequence, from 0.02 in fr1 to 0.23 in fr5 . This result contrasts with the behavior observed for conventional D-A-based TADF molecular architectures [12] . Inspired by this finding, we applied the multiple charge resonance strategy to design in silico new TADF chromophores based on π-extended B-doped and N-doped nanographenes (Fig. 3a ). The results reported in Fig. 3b confirm the trends observed for the fragments in Fig. 2 , i.e., reduced Δ E ST (as supported by the Zero Field Splitting calculations, see Supplementary Table 4 ) and enhanced f osc . In the largest compound investigated, 6 , the singlet and triplet excitations are found to be quasi-degenerate (Δ E ST ~3 meV), yet the singlet f osc is as large as 1.0. 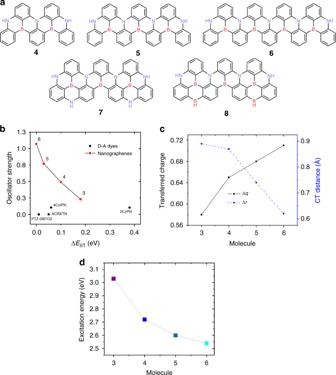Fig. 3 Excited state properties for the designed boron-doped and nitrogen-doped π-extended nanographenes.aChemical structures of engineered molecules4–8. Compound3coincides withfr5in Fig.2a.bOscillator strength,fosc, as a function of ∆ESTfor3–6(red squares) against conventional D-A reference TADF emitters (black dots, see chemical structures in Supplementary Fig.3).cTransferred charge (in |e|) and CT distance (Å), as computed for molecules3–6.dEmission energies and respective colors for3–6 Moreover, as all investigated molecules have a rigid backbone with small (intramolecular) nuclear reorganization energies (Supplementary Table 3 ), we expect these give rise to narrow linewidth and pure color emission. It is important to stress that the increment in f osc is not solely caused by the increase of the number of π-electrons but, instead, occurs primarily through extended delocalization of the wavefunction and increased polarizability along the main-axis of the molecules. Fig. 3 Excited state properties for the designed boron-doped and nitrogen-doped π-extended nanographenes. a Chemical structures of engineered molecules 4–8 . Compound 3 coincides with fr5 in Fig. 2a . b Oscillator strength, f osc , as a function of ∆ E ST for 3 – 6 (red squares) against conventional D-A reference TADF emitters (black dots, see chemical structures in Supplementary Fig. 3 ). c Transferred charge (in |e|) and CT distance (Å), as computed for molecules 3 – 6 . d Emission energies and respective colors for 3 – 6 Full size image Additional insights into this unexpected behavior can be gained from a detailed analysis of the singlet excited-state wavefunctions, in particular of the following two metrics that assess the relative electron-hole quasi-particles: the electron-hole separation (∆ r ) and the amount of charge transferred (∆ q ). Figure 3c points to a picture where the low-lying singlet excited state undergoes substantial reshuffling of the electronic density (large ∆ q values) but over short distances (small ∆ r values). Besides, these characteristics get more pronounced as the ribbons grow longer: ∆ r decreases from 0.9 to 0.6 Å when going from 3 to 6 , while ∆ q increases from 0.58 |e| in 3 up to 0.71 |e| in 6 . The resulting ‘short-range/local CT’ states feature both high electron-hole wavefunction overlaps and small exchange interactions, turning into high f osc and low Δ E ST values for the DABNA core building block. In addition, ‘long-range’ π-conjugation along ribbons 3–6 translates into electronic excitations with extended delocalization and hence increased polarizability and radiative decay rates. While none of these effects is surprising when taken separately, it is the combination of short-range charge separation and long-range electronic delocalization that makes these molecules unique. We believe this is a real breakthrough as most of the low Δ E ST TADF molecules reported so far are characterized by very low f osc and radiative decay rates. This is exemplified by the comparison of compounds 3–6 with selected D-A TADF reference molecules, for which f osc and Δ E ST calculated at a similar level of theory (Fig. 3b and Supplementary Table 2 ) are concurrently small, in line with their ∆ r values larger than the 1.5–2.0 Å criterion usually set to discriminate CT excitations [18] that we reported previously [12] . Finally, besides the beneficial effect on Δ E ST and f osc , increased delocalization along the series 3 – 6 expectedly produces a spectral red-shift of the lowest singlet excitation, thereby allowing for variations of the emission color from blue to green as a function of the molecular size (Fig. 3d ). Further tuning of the emission wavelength can be achieved, for instance by introducing an excess amount of N-atoms or B-atoms into the conjugated plane. For the sake of illustration, we designed two other molecules, 7 and 8 , based on 5 . These chromophores essentially retain the properties of the parent molecule in terms of Δ E ST and f osc (see Supplementary Table 3 ), however, they possess emission wavelengths blue-shifted to 2.85 eV (435 nm, deep blue, 7 ) and red-shifted to 2.1 eV (590 nm, yellow, 8 ) compared to 5 . To conclude, using highly correlated wavefunction-based methods, we have elucidated the origin for the reduced singlet-triplet gap in the boron-centered azatriangulene molecules originally reported by Hatakeyama et al. as resulting from a local alternating rearrangement of the electronic density upon excitation. We have further shown that this is compatible with high absorption and emission extinction coefficients and we have proposed a strategy, based on promoting short-range charge-transfer in π-extended chromophores, as a way to simultaneously optimize RISC and radiative decay rates. This approach has been successfully applied to the design of TADF molecules with: (i) close-to-resonant lowest singlet and triplet excited states; (ii) large singlet radiative decay rates; (iii) tunable and expected pure color singlet emission. We hope our theoretical work will catalyze the synthesis and trigger the characterization of a new generation of TADF molecules with unprecedented electroluminescence quantum efficiencies. Computational details The SCS-CC2 calculations were performed by the TURBOMOLE 6.5 software [19] using the spin-adapted formulation of the linear response theory and the def2-TZVP basis set [20] . The TD-DFT calculations were carried out using the def2-TZVP basis set. The TD-DFT calculations together with the respective analysis, were performed with the ORCA 4.0.1.2 software [21] .